Direct transfer of tri- and di-fluoroethanol units enabled by radical activation of organosilicon reagents Trifluoroethanol and difluoroethanol units are important motifs in bioactive molecules, but the methods to direct incorporate these units are limited. Herein, we report two organosilicon reagents for the transfer of trifluoroethanol and difluoroethanol units into molecules. Through intramolecular C-Si bond activation by alkoxyl radicals, these reagents were applied in allylation, alkylation and alkenylation reactions, enabling efficient synthesis of various tri(di)fluoromethyl group substituted alcohols. The broad applicability and general utility of the approach are highlighted by late-stage introduction of these fluoroalkyl groups to complex molecules, and the synthesis of antitumor agent Z and its difluoromethyl analog Z′. Fluorine incorporation has been a routine strategy for the design of new drugs and materials, because it can often improve the chemical, physical, and/or biological properties of organic molecules [1] , [2] . Fluoroalkylsilicon reagents, such as TMSCF 3 (Rupert–Prakash reagent), TMSCF 2 H, and others are widely used reagents in the synthesis of organofluorine compounds [3] . Among various fluorine-containing molecules, the secondary fluoroalkyl alcohols are of particular importance; monoamine oxidase A inhibitor Befloxatone [4] and antitumor agent Z [5] are examples of bioactive molecules containing trifluoroethanol motif (Fig. 1a ). Anionic activation of C–Si bond of fluoroalkylsilicon reagents by Lewis bases is a powerful method to transfer α-fluoro carbanions into aldehydes, affording fluoroalkyl alcohol products (Fig. 1b ) [6] , [7] , [8] . However, we enviosioned that the development of organosilicon reagents such as 1a and 2a which allows direct transfer of trifluoroethanol and difluoroethanol into organic molecules would represent a conceptually different means to construct fluoroalkyl alcohols (Fig. 1c ). Actually, the synthetic chemistry based on carbonyl group (Fig. 1b ) possesses some limitations: (1) many aldehydes are not stable and/or need multistep synthesis [9] , [10] ; (2) it is hard to control the regioselectivity when there are more than one aldehyde sites in the same molecule. Moreover, the design and synthesis of pharmacuticals call for strategies to incorporate important structural motifs at late-stage, because this will aviod de novo synthesis [11] , [12] . Fig. 1: Secondary fluoroalkyl alcohol synthesis with fluorinated organosilicon reagents. a Representative bioactive molecules containing trifluoroethanol unit. b Organosilicon reagents has been used in the synthesis for secondary fluoroalkyl alcohols via α -fluoro carbanions transfer. c Organosilicon reagents for direct transfer of tri(di)fluoroethanol units via radical activation strategy is developed (this work). Full size image Herein, we report two fluoroalkylsilicon reagents 1a and 2a . Through intramolecular C–Si bond activation by alkoxyl radicals [13] , [14] , [15] , [16] , [17] , [18] , [19] , these developed β-fluorinated organosilicon reagents were successfully applied in radical allylation, alkylation, and alkenylation reactions, enabling efficient synthesis of a variety of fluoroalkyl group substituted alcohols (Fig. 1c ). The broad applicability and general utility of the approach are highlighted by late-stage introduction of fluoroalkyl groups to complex molecules, such as the derivatives from biologically active naturally occuring epiandrosterone, cholesterol, testosterone, diosgenin, vitamin E, estrone, and (8α)-estradiol, and the synthesis of antitumor agent Z and its difluoromethyl analog Z′ . Moreover, our radical reactions show conjunctive group tolerance to that of the traditional nucleophilic fluoroalkylation reactions with α-fluoro carbanions [3] , [20] , [21] (Radical reactions often show different reactivity to the anionic reactions, see refs. [20] , [21] ). Preparation of reagents 1a and 2a The fluoroalkyl group transfer reagents 1a and 2a were easily synthesized in three steps (Fig. 2 ). Following the reported procedure [22] , with commercially available inexpensive trifluoroethanol 3 as starting material, we prepared difluorinated enol silyl ether 4 in 84% yield. Electrophilic fluorination of compound 4 with Selectfluor afforded trifluoroacetylsilane 5 in 82% yield. Reagent 1a was then synthesized in 86% yield through reduction of acylsilane 5 with NaBH 4 . We also prepared different silyl group-substituted compounds 1b – 1d through similar procedures as 1a in good yield (for details, see Supplementary Figs. 2 – 4 ). It is worthy to note that trifluoroacetyltriphenylsilane (precursor to 1d ) can be synthesized directly from the reaction of Ph 3 SiLi and (CF 3 CO) 2 O in one step [23] . The difluoroacetylsilane 6 was easily prepared in 79% yield through the hydrolysis of enol silyl ether 4 under acidic conditions. Reduction of compound 6 delivered difluoromethyl containing reagent 2a in 88% yield. Fig. 2: Preparation of fluoroalkyl group transfer reagents 1a and 2a. With commercially available 3 , reagents 1a and 2a are easily prepared in three steps. Full size image Attempts for anionic activation and design of radical activation With reagent 1a in hand, we investigated the substitution reaction with allylic sulfone 7a as model substrate. Firstly, we tried anionic activation strategy which has been widely used in the C–Si bond cleavage for the fluoroalkyl transfer reactions [6] , [7] , [8] . Common activators such as TBAF, CsF, KF, t -BuOK were tried, but no substitution product 8a or 9a was observed, albeit full conversion of compound 1a was observed (Fig. 3a ). The decomposition of compound 1a could be explained by the facile fluoride elimination of β-fluoro carbanions (Fig. 3b ) [23] , [24] , [25] . For example, Xu and coworkers reported the reaction of trifluoroacetyltriphenylsilane with Grignard reagents, but no desired trifluoromethylated alcohols were obtained. Instead, 2,2-difluoro enol silyl ethers were formed through nucleophilic addition, anion Brook rearrangment, and fluoride elimination processes [23] . It is known that fluorine radical possesses much higher energy than fluorine anion does (Fluorine possesses high electron affinity (3.448 eV), extreme ionization energy (17.418 eV), see ref 1a, pp 5–8). Therefore, we envisioned that in-situ generated carbon radical from alkoxyl radicals should not prefer β-F elimination. Consequently, they could be trapped by radical acceptors to generate trifluoroethanol transfer products (Fig. 3b ). Fig. 3: Attempts for anionic activation and design of radical activation. a Attempts of anionic activation for trifluoroethanol transfer failed. b Facile β-F anion elimination might be the reason of the failure of anionic activation strategy; we designed a radical activation strategy based on the proposal that it is difficult to eliminate high-energy fluorine radical. Full size image Identification of conditions for radical C–Si activation With this idea in mind, we investigated a variety of conditions which could generate alkoxyl radicals (for details, see Supplementary Tables 1 – 3 ). 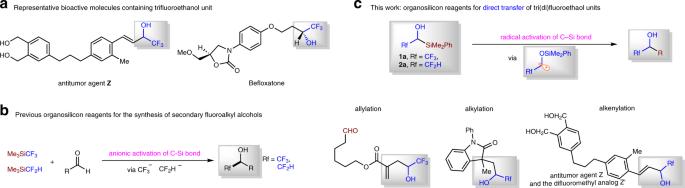Fig. 1: Secondary fluoroalkyl alcohol synthesis with fluorinated organosilicon reagents. aRepresentative bioactive molecules containing trifluoroethanol unit.bOrganosilicon reagents has been used in the synthesis for secondary fluoroalkyl alcohols viaα-fluoro carbanions transfer.cOrganosilicon reagents for direct transfer of tri(di)fluoroethanol units via radical activation strategy is developed (this work). After extensive screening, we found that employing 2 equivalent of Mn(OAc) 3 ·2H 2 O as oxidant, DCM as solvent led to allylation product in 68% yield (Table 1 , entry 1). Further investigation revealed that with 20 mol% of Mn(OAc) 3 ·2H 2 O as catalyst and 2.5 equivalent of TBPB as oxidant, product 8 was given in 61% yield (Table 1 , entry 2). Changing the silyl group from SiMe 2 Ph to SiMePh 2 or SiEt 3 resulted in only slightly decreased yield, but the SiPh 3 -substituted reagent 1d afforded much lower yield (Table 1 , entries 3–5). It was found that Mn(OAc) 2 ·4H 2 O can also be used as catalyst (Table 1 , entry 6). When 20 mol% of Mn(OAc) 2 ·4H 2 O was used, 1a / 7a /TBPB is 1/2/2.5, a yield of 81% can be detected by 19 F NMR with PhCF 3 as an internal standard (Table 1 , entry 7). Control experiments verified that both Mn(II) catalyst and oxidant are necessary for the success of the reaction (Table 1 , entries 8 and 9). When 2,2,2-trifluoroethanol was used instead of compound 1a in our reaction, no conversion of trifluoroethanol was observed (Table 1 , entry 10). The high BDE of C–H bond (409 kJ/mol) in trifluoroethanol might be one of the reasons for the difficulty in the generation of desired radical directly from trifluoroethanol under mild conditions [26] , [27] , [28] , [29] (There are limited reports on the generation of carbon radicals from trifluoroethanol under harsh conditions, see refs. [27] , [28] , [29] ). The attempt to use Smith’s condition [19] to achieve the reaction between 1a and 7a failed to afford any amount of product 8a or 9a , highlighting the influence of CF 3 group on the reactivity of reagent 1a . Table 1 Reaction optimization a . Full size table Synthesis of α-trifluoromethylated homoallylic alcohols We next explored the scope of the allylic substitution reaction (Fig. 4 ). Both Mn(OAc) 3 ·2H 2 O and Mn(OAc) 2 ·4H 2 O are efficient catalysts for the transformation. When TBAF was used to quench the reaction, the silyl ether was converted to alcohol in one pot, and compound 9a was isolated in 62% yield. It was found that a variety of allylic sulfones [30] , [31] , [32] , [33] , [34] bearing different groups could be used as the radical acceptors, affording the α-CF 3 -substituted homoallylic alcohols 9a – 9ap in 40–83% yields. This reaction can be scaled up, and a yield of 65% was obtained for compound 9c (1.25 g isolated), and the sulfone 7c was recovered in 61% yield after silica gel chromatography. It is worth noting that the current allylation protocol can tolerate many functional groups. The Csp 2 –F, Csp 2 –Cl, Csp 2 –Br, Csp 2 –I bond can be kept after the reaction, affording compounds 9d – 9i , 9u , and 9v in 56–83% yields. Moreover, allylic bromide can also be tolerated ( 9j , 48% yield). These functional groups are well-known convertible motifs under transition metal-mediated/catalyzed reactions. Electron donating OMe group, electron withdrawing groups, such as NO 2 , CN can also be tolerated, affording compounds 9k – 9m in 68–80% yields. Electron-rich heterocyclic groups, such as furyl and thienyl are also be tolerated ( 9n , 80% yield; 9o , 82% yield). Naphthyl-substituted product was also successfully made via the Mn-catalyzed substitution reaction, affording alcohol 9p in 72% yield. A variety of alkyl ethers and benzylic alcohol-derived esters are tolerated under the current oxidation conditions, and alcohols 9q – 9w were obtained in 56–73% yields. Not only ester-substituted and ketone-substituted allylic sulfones, but also amide, sulfone, phenyl, and alkyl groups-substituted allylic sulfones can be applied in the current substitution process, affording corresponding α-CF 3 -substituted homoallylic alcohols ( 9z – 9ad , 40–72% yields). 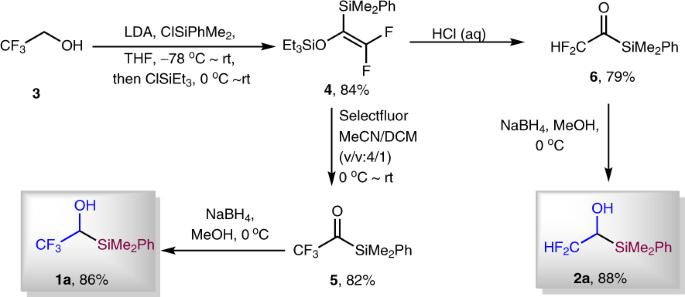Fig. 2: Preparation of fluoroalkyl group transfer reagents 1a and 2a. With commercially available3, reagents1aand2aare easily prepared in three steps. Moreover, this substitution process is compatible with many base-sensitive functionality, such as primary alcohol ( 9af , 45% yield), alkyl aldehyde ( 9ag , 46% yield), alkyl ketone ( 9ah , 62% yield; 9aj , 59% yield; 9al , 63% yield; 9ao , 46% yield). It is worthy to note that the above-mentioned aldehyde and ketone-containing products are challenging to be synthesized by methods based on these functional groups [3] . In addition, the current radical allylic substitution can be applied in the functionalization of complex molecules, such as the derivatives from biologically active naturally occuring epiandrosterone, cholesterol, testosterone, diosgenin, vitamin E, estrone, and (8α)-estradiol, affording corresponding alcohols 9ai – 9ap in 46–75% yields. Fig. 4: Scope for the allylation of reagent 1a. a 1a/ 7 = 1/3, b 1a / 7 = 1/2, and c Mn(OAc) 3 ·2H 2 O was used instead of Mn(OAc) 2 ·4H 2 O. d 2 equivalent of Mn(OAc) 3 ·2H 2 O was used without TBPB. e Instead of TBAF, water was used to quench the reaction. Full size image Synthesis of α-trifluoromethylated alkyl alcohols After achieving the radical C–Si bond activation to access α-trifluoromethylated homoallylic alcohols, we wondered whether the same strategy can be applied in double functionalization of alkenes to prepare α-trifluoromethylated alkyl alcohols. Acryl amides 10 were chosen to test the possibility [35] , [36] , [37] , [38] . To our delight, under Mn(II)/TBPB conditions, various acryl amides can be converted to corresponding trifluoromethylated alcohols 11 in 63–91% yield (Fig. 5 ). Me, Ph, and Bn groups on the N of amides do not affect the reaction. The reaction tolerates halides, such as F and Cl. Both electron-donating OMe and electron-withdrawing CO 2 Me on the arenes were maintained after the reaction. It is worthy to note that compounds 11 are difficult to be synthesized through the nucleophilic trifluoromethylation reaction of aldehydes with TMSCF 3 , because the aldehydes themselves need multistep synthesis [10] . Fig. 5: Synthesis of α-trifluoromethylated alkyl alcohols. All reactions were run under the standard conditions with 1a/10 = 1/2. Full size image Synthesis of α-trifluoromethylated allylic alcohols Allylic alcohols are important synthetic intermediates for a variety of transformations. Moreover, fluorinated compounds possess unique chemical, physical, and biological properties. Therefore, the development of one step synthesis of α-trifluoromethylated allylic alcohols from readily available starting materials are highly desired. Previous methods to prepare α-trifluoromethylated allylic alcohols mainly rely on nucleophilic trifluoromethylation of α,β-unsaturated aldehydes [39] , [40] , [41] , [42] , [43] . α,β-Unsaturated carboxylic acids are easy to be synthesized and many of them are commercially available. Moreover, they are more stable under atmosphere than corresponding α,β-unsaturated aldehydes. They have been used in the decarboxylative trifluoromethylation reactions for the synthesis of CF 3 -substituted alkenes [44] , [45] . Encouraged by the success of synthesizing homoallylic and alkyl alcohols with 1a as reagent under the radical C–Si bond activation conditions, we studied the reaction between 1a and acids 12 to prepare α-trifluoromethylated allylic alcohols (Fig. 6 ). The reaction conditions are slightly different from the above allylation and alkylation reactions: (1) both hexane and DCM could be used as solvent; (2) the desilylation step was performed under lower temperature (−10 vs. 5 °C) to avoid side reactions. It can be found from Fig. 7 that various α,β-unsaturated carboxylic acids containing F, Cl, Br, MeO, BnO, and CF 3 substituents were successfully converted to corresponding α-trifluoromethylated allylic alcohols in 51–75% yield. To the best of our knowledge, there has been no report on the synthesis of α-trifluoromethylated allylic alcohols with unsaturated carboxylic acids before this work. Fig. 6: Synthesis of α-trifluoromethylated allylic alcohols. a Reactions were run under standard conditions with 1a / 12 = 1/2. b DCM was used as solvent instead of hexanes. Full size image Fig. 7: Synthesis of α-difluoromethylated alcohols. a Mn(OAc) 3 ·2H 2 O (20 mol%) was used as catalyst. b Mn(OAc) 2 ·4H 2 O (20 mol%) was used as catalyst. c DCM (0.1 M) was used as solvent. d Hexane (0.4 M) was used as solvent. e t = 18 h and f t = 14 h. Full size image Radical C–Si activation for difluoroethanol unit transfer Difluoromethyl group (CF 2 H) is isopolar and isosteric to an SH or OH group, and can also behave as a hydrogen donor through hydrogen bonding [46] , [47] . Therefore, difluoromethylated compounds are strong candidate for drugs. There are examples showing that the CF 2 H-containing compounds exhibit higher bioactivity than their CF 3 -containing counterparts [48] , [49] . Encouraged by the above success of radical C–Si bond activation to access trifluoromethylated allylic, alkyl, and alkenyl alcohols, we extended the strategy to directly transfer 2,2-difluoroethanol to organic molecules with reagent 2a (Fig. 7 ). To the best of our knowledge, there has been no report of the synthetic application of carbon radical from 2,2-difuoroethanol. Under the similar reaction conditions as that of 1a , with allylic sulfones as substrates, difluoromethylated homoallylic alcohols 14a – 14c were prepared in 66–80% yield. Late-stage functionalization of two complex molecules are also successful; 14d and 14e were isolated in 83% and 67% yield, respectively. The reactions of acryl amides performed well, affording 14f – 14i in 76–82% yield. Ph, Bn, and Me groups on the N atom were tolerated; both electron-withdrawing CO 2 Me and electron-donating OMe groups on the aromatic ring were maintained after the reactions. Three examples of α,β-unsaturated carboxylic acids demonstrated the utility of synthesis of difluoromethyl group-substituted allylic alcohols 14j – 14l in synthetically useful yield. Synthesis of antitumor agent Z and its difluoromethyl analog Z′ After achieving the direct transfer of 2,2,2-trifluoroethanol and 2,2-difluoroethanol to simple α,β-unsaturated carboxylic acids, we tested whether our methodology can be applied in the synthesis of antitumor agent Z (Fig. 8 ) [5] . Starting from known compound 15 [5] , the protection of phenol afforded compound 16 in 97% yield. α,β-Unsaturated carboxylic acid 17 was then synthesized in 76% yield after Heck reaction and selective hydrolysis of the ester. The radical reactions performed well under our standard conditions, affording compounds 18 and 19 in 71% yield and 69% yield, respectively. Hydrolysis of the esters afforded the final product Z and Z′ in 94% and 89% yield, respectively. Fig. 8: Synthesis of antitumor agent Z and its difluoromethyl analog Z′. Tf 2 O trifluoromethanesulfonic anhydride, DPPP bis(diphenylphosphino)propane, TFA trifluoroacetic acid, DIBAL-H diisobutylaluminum hydride. Full size image Mechanism of the study The radical inhibition experiments revealed that addition of 1 equiv. of TEMPO or BHT can completely inhibit the allylation reaction, albeit more than 60% of compound 3a were consumed in both cases (Fig. 9a ). In addition, compound 21 was detected by HRMS when TEMPO was added into the reaction (for details, see Supporting Information). Therefore, radical process might be involved in current substitution reaction. Our investigation revealed that Mn(OAc) 3 ·2H 2 O is able to mediate the reaction without external oxidant, but Mn(OAc) 2 ·4H 2 O cannot mediate the reaction without TBPB (Table 1 , entries 1 and 8). Based on these results, we propose a possible mechanism as shown in Fig. 9b . Ligand exchange between Mn(III) species and alcohol 1a might generate intermediate I , which undergoes homolysis to produce alkoxyl radical II and Mn(II) intermediate [50] , [51] , [52] , [53] . Carbon radical III would be generated through Brook rearrangement, and then undergo further reaction to generate product IV . Mn(III) catalyst is likely to be regenerated by the oxidation of Mn(II) by TBPB. The alcohol product V would be generated after the desilylation step. It is worthy to note that the reaction pathways in the allylation, alkylation, and alkenylation reactions are probably different (for the proposed possibilities, see Supplementary Figs. 13 – 15 ). 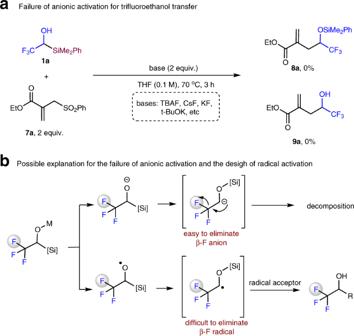Fig. 3: Attempts for anionic activation and design of radical activation. aAttempts of anionic activation for trifluoroethanol transfer failed.bFacile β-F anion elimination might be the reason of the failure of anionic activation strategy; we designed a radical activation strategy based on the proposal that it is difficult to eliminate high-energy fluorine radical. As for the nature of radical III , we propose that they are nucleophilic radicals. The following facts support this proposal: (1) the reaction partners in the above three kinds of reactions are electron-deficient olefins; (2) more electron-deficient substrate afforded higher yield (for example, Fig. 5 , 9ac , 43% yield; 9ae , 70% yield); (3) the carbon radical generated from trifluoroethanol under γ-ray irradiation could add to highly electrophilic hexafluoro-2-butyne [27] . Fig. 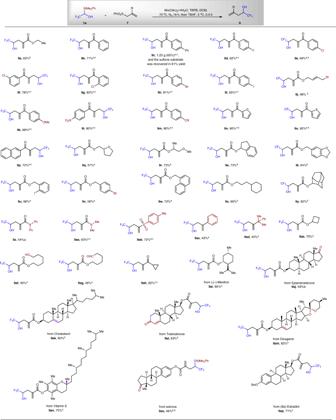Fig. 4: Scope for the allylation of reagent 1a. a1a/7= 1/3,b1a/7= 1/2, andcMn(OAc)3·2H2O was used instead of Mn(OAc)2·4H2O.d2 equivalent of Mn(OAc)3·2H2O was used without TBPB.eInstead of TBAF, water was used to quench the reaction. 9: Radical inhibition experiments and proposed mechanism. a TEMPO and BHT efficiently inhibited the allylation reaction, supporting radical process might be involved. b A plausible mechanism is proposed. Full size image In conclusion, we have developed two fluorinated organosilicon reagents, which were used in direct transfer of trifluoroethanol and difluoroethanol units into organic molecules. A radical C–Si bond activation strategy was developed to solve the problem of β-fluorine elimination in anionic activation methods. Upon intramolecular activation of C–Si bond by alkoxyl radicals, the β-fluoro carbon radicals were generated and participated in efficient allylation, alkylation, and alkenylation reactions, enabling efficient synthesis of numerous fluoroalkyl alcohols. The broad applicability and general utility of the approach are highlighted by late-stage introduction of fluoroalkyl groups to complex molecules and the synthesis of antitumor agent Z and its difluoromethyl analog Z′ . Further application of the radical C–Si bond activation of organosilicon reagents are underway in our lab. Typical synthesis of compound 9 Under N 2 atmosphere, to a dried 10 mL Schlenk tube equipped with a magnetic stir bar containing Mn(OAc) 2 ·4H 2 O (14.7 mg, 0.06 mmol, 20 mol%) was added DCM (3 mL, 0.1 M), 1a (70.2 mg, 0.3 mmol), 7a (152.4 mg, 0.6 mmol, 2.0 equiv. ), and TBPB (145.7 mg, 0.75 mmol, 2.5 equiv.) sequentially. The tube was sealed, and the resulting mixture was kept stirring at 70 °C in a heating block for 18 h. The mixture was then cooled to 5 °C with ice bath, TBAF (1.0 M in THF, 0.36 mL, 0.36 mmol, 1.2 equiv.) 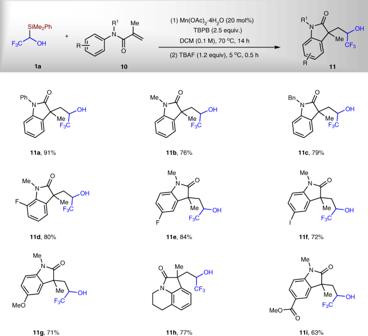Fig. 5: Synthesis of α-trifluoromethylated alkyl alcohols. All reactions were run under the standard conditions with1a/10= 1/2. 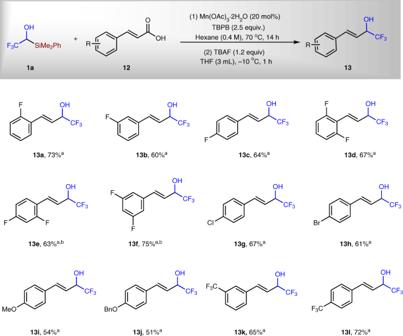Fig. 6: Synthesis of α-trifluoromethylated allylic alcohols. aReactions were run under standard conditions with1a/12= 1/2.bDCM was used as solvent instead of hexanes. 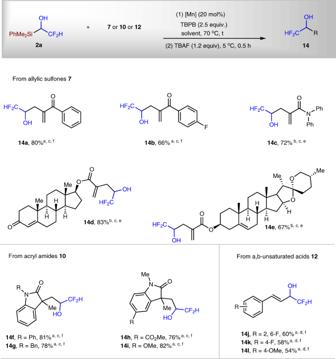Fig. 7: Synthesis of α-difluoromethylated alcohols. aMn(OAc)3·2H2O (20 mol%) was used as catalyst.bMn(OAc)2·4H2O (20 mol%) was used as catalyst.cDCM (0.1 M) was used as solvent.dHexane (0.4 M) was used as solvent.et= 18 h andft= 14 h. 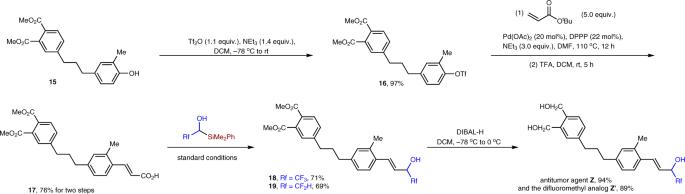Fig. 8: Synthesis of antitumor agent Z and its difluoromethyl analog Z′. Tf2O trifluoromethanesulfonic anhydride, DPPP bis(diphenylphosphino)propane, TFA trifluoroacetic acid, DIBAL-H diisobutylaluminum hydride. 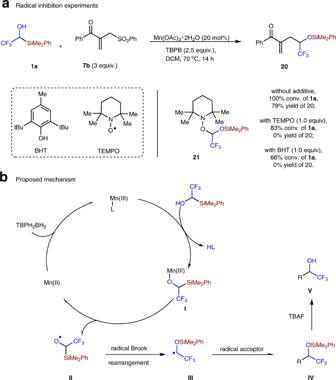Fig. 9: Radical inhibition experiments and proposed mechanism. aTEMPO and BHT efficiently inhibited the allylation reaction, supporting radical process might be involved.bA plausible mechanism is proposed. was added and the resulting mixture was stirred at 5 °C for 0.5 h. The reaction mixture was quenched with water (2 mL), extracted with DCM (3 × 10 mL) and organic phase was combined and washed with brine, dried over Na 2 SO 4 , concentrated under reduced pressure. The crude product was purified with column chromatography on silica gel (200–300 mesh) and PE/EA (20/1–10/1, v/v) as eluent to afford 40.0 mg of compound 9a as a colorless oil (62% yield).